Quantum nuclear dynamics in the photophysics of diamondoids The unusual electronic properties of diamondoids, the nanoscale relatives of diamond, make them attractive for applications ranging from drug delivery to field emission displays. Identifying the fundamental origin of these properties has proven highly challenging, with even the most advanced quantum many-body calculations unable to reproduce measurements of a quantity as ubiquitous as the optical gap. Here, by combining first-principles calculations and Importance Sampling Monte Carlo methods, we show that the quantum dynamics of carbon nuclei is key to understanding the electronic and optical properties of diamondoids. Quantum nuclear effects dramatically modify the absorption lineshapes and renormalize the optical gaps. These findings allow us to formulate a complete theory of optical absorption in diamondoids, and establish the universal role of quantum nuclear dynamics in nanodiamond across the length scales. The smallest diamondoid is a cycloalkane with formula C 10 H 16 named adamantane. Like in the diamond lattice, the carbon atoms of adamantane are sp 3 bonded to form a cage [2] . Conceptually, the entire diamondoid series is generated by fusing adamantane cages together, with two cages corresponding to diamantane C 14 H 20 and three cages to triamantane C 18 H 24 . The structures of these so-called basic diamondoids are shown in Fig. 1a . Further increasing the number of cages generates the higher diamondoids, which exhibit multiple isomers for a given number of cages. 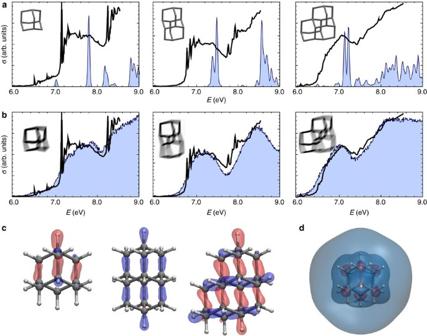Figure 1: Optical absorption spectra and structural models of the basic diamondoids. (a) Absorption spectra of adamantane, diamantane and triamantane (left to right), calculated with the nuclei clamped to their equilibrium positions (blue areas) compared with the experimental spectra reported in Landtet al.24(black lines). The structural model of each diamondoid is also shown. (b) Absorption spectra calculated with nuclear dynamics included using equation (1) (blue areas) again compared with the experimental data of Landtet al.24(black lines; the fuzzy models are a pictorial representation of the quantum nature of the nuclei). (c) Ball-and-stick models and isodensity surfaces of the HOMOs of adamantane, diamantane and triamantane. (d) Isodensity surface of the LUMO of adamantane. Figure 1: Optical absorption spectra and structural models of the basic diamondoids. ( a ) Absorption spectra of adamantane, diamantane and triamantane (left to right), calculated with the nuclei clamped to their equilibrium positions (blue areas) compared with the experimental spectra reported in Landt et al. [24] (black lines). The structural model of each diamondoid is also shown. ( b ) Absorption spectra calculated with nuclear dynamics included using equation (1) (blue areas) again compared with the experimental data of Landt et al. [24] (black lines; the fuzzy models are a pictorial representation of the quantum nature of the nuclei). ( c ) Ball-and-stick models and isodensity surfaces of the HOMOs of adamantane, diamantane and triamantane. ( d ) Isodensity surface of the LUMO of adamantane. Full size image Recently, the discovery of the higher diamondoids in oil and the availability of kilograms of the basic diamondoids [3] have ignited interest in the technological applications of these systems. Diamondoids are biocompatible and ultrahard, therefore ideally suited for applications in drug delivery and nanolubrication [4] , [5] . In organic electronics, they can be used as monochromatic electron emitters owing to their negative electron affinity [6] , [7] , and as fluorescent markers, single-photon sources and nanoscale magnetic sensors using colour centres [8] , [9] . At a more fundamental level, diamondoids constitute ideal test systems for theories of the electronic structure of carbon nanomaterials, and in particular for exploring the interplay between electronic and nuclear dynamics. The absence of p electrons in the core of C atoms leads to the valence 2 p electrons lying very close to the nuclei, thereby enhancing their coupling to the nuclear potential [10] , [11] . Owing to this effect and to the light nuclear mass, one can expect a strong electron–phonon coupling in diamondoids, similar to other carbon allotropes like nanotubes [12] , [13] , diamond [14] , [15] , graphite and graphene [16] , graphane [17] , polymers [18] and fullerenes [19] . In line with this expectation, electron–vibration interactions have been invoked to explain rapid electron thermalization in diamondoid monolayers [20] and the nodal structure of scanning tunnelling microscopy maps [21] . The notion that nuclear dynamics may have an important role in the optical properties of diamondoids is understood intuitively by inspecting their electronic wavefunctions in Fig. 1c . As the highest occupied molecular orbitals (HOMOs) are localized in between C–C bonds, their energy is sensitive to changes in the interatomic bond lengths arising from the motion of the C nuclei. On the other hand, the lowest unoccupied molecular orbitals (LUMOs, shown in Fig. 1d for adamantane) are Rydberg states, which wrap around the diamondoid surface, and are sensitive to the collective motion of the H atoms [21] . In this work, we demonstrate the remarkable role played by nuclear quantum motion in the fundamental photophysics of the diamondoids. Previous many-body Quantum Monte Carlo calculations [7] , [22] have found the onset of optical absorption to be almost an electronvolt higher than measured in experiments, and it has been suggested that vibronic effects may be responsible for the discrepancy [22] . Here, we combine first-principles calculations with Monte Carlo integration techniques to show that not only does the nuclear motion substantially renormalize the calculated optical gaps but also that vibronic couplings dramatically modify the absorption lineshapes, even at zero temperature. Our results highlight the crucial importance of including quantum nuclear effects in the ab initio modelling of carbon-based nanomaterials. Optical absorption with clamped nuclei The optical absorption spectra of adamantane, diamantane and triamantane, calculated under the standard approximation that the nuclei are clamped to their equilibrium positions, are shown as the blue areas in Fig. 1a . These calculations were performed within the local-density approximation to density-functional theory (DFT) using the Quantum ESPRESSO software distribution [23] , with a common scissor correction employed as a remedy for the DFT band gap problem ( Supplementary Note 1 ). The use of more refined time-dependent DFT calculations yields essentially identical results ( Supplementary Fig. S1 ). A comparison between the clamped-nuclei calculations and the measured spectra [24] given by the black lines in Fig. 1a reveals a dramatic failure of the standard theory. Although the calculations display rather sharp absorption peaks, the experimental spectra are broad and featureless, apart from some fine structure in the cases of adamantane and diamantane. In the following, we demonstrate that this severe discrepancy originates from the neglect of quantum nuclear dynamics, and that only by explicitly including nuclear wavefunctions in the theory can quantitative agreement with experiment be obtained. Semiclassical Franck–Condon description of quantum nuclei The experimental spectra in Fig. 1a exhibit two characteristic energy scales, one of the order of electronvolts and the other of the order of tens of millielectronvolts. We propose that these energy scales are to be associated with electronic and nuclear dynamics, respectively, and can be addressed separately through a multiscale approach. For the electronic energy scale, we are not interested in resolving individual quantum nuclear states, therefore we can calculate the absorption cross-section σ ( ω ) using the semiclassical Franck–Condon approximation [25] , [26] , [27] : Here α is the fine structure constant, ħ the Planck constant, R stands for the entire set of (3 N −6) nuclear coordinates ( N being the number of nuclei in the system), and r stands for the electronic coordinates. The electronic states Ψ n ( r ; R ) with energies E n ( R ) are obtained with nuclei clamped in the configuration R , and Φ n ,ν ( R ) represents a (3 N −6)-dimensional nuclear wavefunction obtained from the potential energy surface E n ( R ), that is, a vibron. Similar to diamond [28] , we find the potential energy surface to be accurately described within the harmonic approximation. The optical matrix elements for photons of energy ħω and polarization are evaluated in the electric-dipole approximation, and the braket stands for an integration over the electronic coordinates. The electron-nuclear wavefunction Ψ 0 Φ 0,0 represents the ground state of the system. Intuitively equation (1) yields the absorption spectrum as a weighted average of the spectra calculated with clamped nuclei over all possible nuclear configurations, where each nuclear configuration is weighted with a probability given by the square modulus of the zero-point wavefunction |Φ 0,0 ( R )| 2 . The calculation of the cross-section in equation (1) is challenging as it requires an integration over 3 N −6 dimensions, for example, 120 dimensions for triamantane. In order to address this challenge, we developed an efficient computational method based on Importance Sampling Monte Carlo (ISMC) integration. In ISMC, an integral is replaced by a weighted average of the integrand, sampled at points randomly selected from a probability distribution called the importance function. By choosing the importance function to be localized in the region of phase space where the integrand is large, it is possible to perform the integration very efficiently [29] . Here we use |Φ 00 ( R )| 2 as the importance function, and generate a random set of nuclear configurations accordingly. Then for each configuration, we perform a DFT calculation to determine both the energies and optical matrix elements. By calculating the latter, we automatically include the Herzberg–Teller effect and properly account for degeneracy in the electronic states. We find the ISMC approach to be extremely efficient in converging lineshapes and energies ( Supplementary Fig. S2 ). As each ISMC step requires only one DFT self-consistent calculation, it is possible to accumulate good statistics (10,000 configurations for each diamondoid, see Methods section). The absorption spectra calculated using equation (1) are shown as the blue regions in Fig. 1b . The calculations reproduce the experimental spectra to an excellent level of accuracy at the electronvolt scale. Comparing these results to the spectra determined at clamped nuclei ( Fig. 1a ) shows that the nuclear motion induces a dramatic broadening of the spectral peaks of up to 1 eV, and additionally a redshift of the absorption threshold as large as 0.6 eV (details below). Vibronic transitions in the Franck–Condon approach Moving to the smaller energy scale, we note that the sharp peaks observed in experiment for adamantane and diamantane are missing in the semiclassical approximation of equation (1). These peaks arise from long-lived Born–Oppenheimer resonances [30] and therefore require an explicit description of the excited vibrational quantum states. We decided to proceed with the Franck–Condon approach [25] , where the absorption cross-section reads: where the sum runs over all the quantum nuclear states, and the energy E n ,ν ( R ) is obtained from E n ( R ) in equation (1) by adding the vibronic contribution corresponding to the state Φ n ,ν . If vibronic contributions are neglected, the above equation reduces to equation (1). Equation (2) describes the optical absorption process as electric-dipole transitions between pairs of Born–Oppenheimer states Ψ n Φ n ,ν , and fully takes into account the final vibronic state. In order to focus on transitions around the absorption edge, we make the standard Condon approximation, that is, we ignore the dependence of the matrix elements and electron energies on the nuclear coordinates, and we determine the potential energy surfaces of the nuclei using the electronic ground state and the first excited state within constrained DFT (see Methods section). The evaluation of the (3 N −6)-dimensional Condon integrals in equation (2) is challenging owing to the combinatorial explosion of the number of final states with increasing photon energy. For example, in the case of adamantane, we count 100 billion available final states within the first eV from the absorption onset. In order to circumvent this difficulty, we restrict the sum over final states to a subset of vibrational modes including up to three-phonon transitions and perform the integrals using ISMC. In this case the importance function is taken to be the zero-point nuclear wavefunction Φ 0,0 ( R ) (see Methods section). This choice is possible as the zero-point wavefunction is nodeless, at variance with fermionic systems where the nodal structure of the ground state provides Quantum Monte Carlo methods with a formidable challenge [31] . 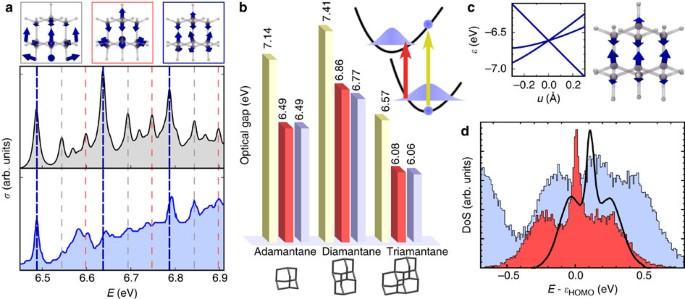Figure 2: Detailed analysis of quantum nuclear effects in the diamondoids. (a) Fine structure in the optical spectrum of adamantane near the absorption onset. The blue line is the experimental spectrum from Landtet al.24, and the black line is the spectrum calculated using equation (2). The coloured vertical dashed lines and corresponding ball-and-stick models with arrows refer to the vibronic progressions discussed in the text. The thick dashed blue lines correspond to the A1mode with energy 149.4 meV. The vibration patterns shown on the top are colour-matched to the corresponding vertical bars. (b) Comparison between measured and calculated optical gaps of diamondoids. Vertical excitations (yellow arrow/bars) cannot explain the measured band gaps (blue bars), while adiabatic excitations (red arrow/bars) are in very good agreement with experiment. (c) Triplet splitting of theT2HOMO of adamantane as a function of theT2C–C stretching mode illustrated by the arrows. (d) ISMC calculation of the density-of-states of adamantane near the HOMO. The energy axis is aligned with the HOMO calculated for nuclei clamped at their equilibrium positions. The red area is obtained by considering only the coupling to theT2modes, the blue area is obtained by considering all vibrational modes. The thick black line corresponds to the valence band top in diamond obtained in Ramírezet al.26using path-integral molecular dynamics. Figure 2a shows the optical cross-section of adamantane calculated using equation (2) near the onset (black line). Our calculations (blue line) are in good agreement with experiment [24] , indicating that the observed fine structure arises from Condon effects. A detailed analysis of the calculated spectrum allows us to rationalize the most prominent spectral features in terms of a series of vibronic peaks at energies multiples of 149.4 meV, accompanied by satellites shifted by 56.2 and 110.2 meV, respectively. The mode at 149.4 meV corresponds to the A 1 stretching vibration of the C atoms in the cage, and the two satellites to A 1 deformations of the C–C–C bridges (see Methods section). The main vibronic series and its satellites are shown as thick and thin vertical bars in Fig. 2a , respectively, and match well the calculated and measured peaks at low energy. This series is also found to account for the fine structures associated with higher electronic transitions in adamantane and for the spectrum of diamantane. Therefore, we find that a simple universal law underpins the vibronic fine structures in the optical spectra of the basic diamondoids. Interestingly, the same C–C stretching mode at the origin of these vibronic features is also responsible for the band gap renormalization of bulk diamond [14] , [15] , and for the superconducting properties of boron-doped diamond [32] . Figure 2: Detailed analysis of quantum nuclear effects in the diamondoids. ( a ) Fine structure in the optical spectrum of adamantane near the absorption onset. The blue line is the experimental spectrum from Landt et al. [24] , and the black line is the spectrum calculated using equation (2). The coloured vertical dashed lines and corresponding ball-and-stick models with arrows refer to the vibronic progressions discussed in the text. The thick dashed blue lines correspond to the A 1 mode with energy 149.4 meV. The vibration patterns shown on the top are colour-matched to the corresponding vertical bars. ( b ) Comparison between measured and calculated optical gaps of diamondoids. Vertical excitations (yellow arrow/bars) cannot explain the measured band gaps (blue bars), while adiabatic excitations (red arrow/bars) are in very good agreement with experiment. ( c ) Triplet splitting of the T 2 HOMO of adamantane as a function of the T 2 C–C stretching mode illustrated by the arrows. ( d ) ISMC calculation of the density-of-states of adamantane near the HOMO. The energy axis is aligned with the HOMO calculated for nuclei clamped at their equilibrium positions. The red area is obtained by considering only the coupling to the T 2 modes, the blue area is obtained by considering all vibrational modes. The thick black line corresponds to the valence band top in diamond obtained in Ramírez et al. [26] using path-integral molecular dynamics. Full size image By combining our calculations for the two energy scales in Figs 1a and 2a , we obtain a complete picture of the optical spectra of adamantane, diamantane and triamantane. In larger diamondoids, the increasing density of vibronic states yields quasicontinuous band-like absorption, such that even for triamantane sharp features are not seen in the optical spectrum. Therefore, starting from triamantane the semiclassical approximation of equation (1) provides an accurate description of the absorption spectrum of diamondoids, explaining the success of its application to the case of bulk diamond [14] , [15] , [27] . We now quantify the effect of nuclear dynamics on the optical gaps of diamondoids. Based on the comparison between theory and experiment in Fig. 2a , we assign the first optical excitation to an adiabatic transition between the two zero-point wavefunctions in the electronic ground and excited states (inset of Fig. 2b ). The adiabatic excitation energy is smaller than for the standard vertical transitions as it includes the effect of structural relaxation and a shift in quantum zero-point energy ( Fig. 2b ). Our calculations yield substantial redshifts of 650, 550 and 490 meV for adamantane, diamantane and triamantane, respectively, reflecting significant structural relaxations upon photoexcitation. Figure 2b shows how, by taking into account the adiabatic nature of the fundamental optical gap in diamondoids, much better agreement with experiment is obtained. Combining our results with the calculations of Marsusi et al. [22] ( Supplementary Note 1 ) reduces the discrepancy between experimental and Quantum Monte Carlo-calculated optical gaps from 0.8 to 0.3 eV. This difference is within the error bar estimated by Marsusi et al. [22] , and is of the order of the difference between DMC data and GW calculations of the ionization potentials [33] . This result identifies the change in quantum nuclear energy upon photoexcitation as the missing physics in previous attempts at explaining the optical properties of diamondoids [7] , [22] , [34] . The redshift of the optical gaps determined here for diamondoids is surprisingly similar to the renormalization of 615–670 meV found in bulk diamond [14] , [15] . This similarity establishes an unexpected connection between the photophysics of the basic diamondoids and bulk diamond, and suggests that zero-point effects are largely consistent among sp 3 carbon materials irrespective of size. Extension to finite temperatures The results shown in Fig. 2b were obtained at zero temperature. In order to extend our analysis to finite temperatures, we calculated the temperature dependence of the redshifts using the semiclassical Allen–Heine theory [35] . The temperature dependence of the single particle eigenvalue E n is given by [36] : where n B, i is the Bose–Einstein factor for the i -th vibrational mode at the temperature T , and E n is evaluated for nuclei clamped at their equilibrium positions. m p is the proton mass. The temperature shifts were obtained by calculating the second derivatives using finite displacements of size along the normal mode coordinates. The shifts of the optical gaps upon heating the diamondoids from 0–300 K were found to be extremely small, 2, 15 and 7 meV for adamantane, diamantane and triamantane, respectively. These figures indicate that the electronic structure of diamondoids is dominated by quantum zero-point effects at all experimentally relevant temperatures. Anomalous Jahn–Teller effect in adamantane The close analogy between the zero-point effects in the end-members of the sp 3 carbon family prompted us to explore other possible links between adamantane and diamond. The HOMO of adamantane is triply degenerate and hence expected to undergo a Jahn–Teller splitting upon photoexcitation [37] . However, different experiments led to contrasting conclusions on the existence of a Jahn–Teller effect in adamantane [38] , [39] . Figure 2c shows how the threefold-degenerate HOMO of adamantane is split into a triplet by the C–C stretching vibrations of T 2 symmetry at 161.2 meV. These vibrations are the ground-state counterparts of the stretching modes responsible for the vibronic series in photoexcited adamantane. An ISMC calculation where only these modes are active shows that the lineshape of the HOMO develops a narrow central peak and two wide sidebands (red shaded region in Fig. 2d ), that is, precisely the spectral fingerprint of the T - t 2 Jahn–Teller coupling [37] . If we now recalculate the lineshape by including the coupling to all the vibrational modes, we find a substantial redistribution of spectral weight, which has the effect of strengthening the sidebands (light blue shaded area of Fig. 2d ) and obscuring the T - t 2 Jahn–Teller fingerprint. The resulting anomalous Jahn–Teller lineshape identified here reconciles previous contrasting interpretations [38] , [39] . Most importantly, the Jahn–Teller signature of adamantane is strikingly similar to that calculated for bulk diamond using path-integral molecular dynamics [27] (black line in Fig. 2d ) showing that the two end-members of the sp 3 carbon family are linked by a universal electron–phonon coupling. Taken all together, our findings outline the first complete theory of optical absorption in the basic diamondoids in quantitative agreement with experiment, and provide compelling evidence for the role of quantum nuclear dynamics in the photophysics of these systems. Given the remarkable similarities between vibronic effects in diamondoids and electron–phonon effects in bulk diamond, it is expected that our results will apply across the length scales to encompass the higher diamondoids and detonation diamonds. As quantum nuclear dynamics is likely to have a role also in other technologically important properties of diamondoids, for example, the transitions rates of single-photon sources [40] , the bandwidth of electron emitters [6] and the spin coherence times of colour centres [41] , there is an urgent need to establish efficient procedures for systematically incorporating nuclear wavefunctions into the first-principles modelling of nanomaterials. DFT calculations All calculations were performed within Kohn–Sham DFT [42] , [43] using the Quantum ESPRESSO software distribution [23] . The exchange and correlation energy was treated using the local-density approximation of Ceperley and Alder as parametrized by Perdew and Zunger (DFT-LDA) [44] , [45] . The valence electron wavefunctions and charge density were expanded in a plane-wave basis set with kinetic energy cutoff of 80 Ry, and the core-valence interaction was taken into account by using norm-conserving pseudopotentials [46] . A Coulomb truncation scheme [47] was employed in order to remove spurious interactions between periodic replicas of the computational cell, and the ground-state geometry of each diamondoid was obtained by minimizing the Hellmann–Feynman forces until they were below 25 meV Å −1 . An empirical scissor correction of 1.21 eV was applied to the unoccupied Kohn–Sham states. The vibrational frequencies were calculated by evaluating the dynamical matrices obtained in finite-difference calculations. Optical absorption spectra at clamped nuclei The optical absorption spectra of the diamondoids with nuclei clamped in their equilibrium positions (blue areas of Fig. 2a ) were obtained from equation (1) by replacing the nuclear wavefunctions with Dirac’s delta functions centred at the equilibrium positions R 0 of the nuclei, and expressing the many-body electronic wavefunction by a single determinant of Kohn–Sham states. Orientational averages were taken using the trace over the Cartesian directions. Supplementary Fig. S1 shows that in the case of the basic diamondoids the scissor-corrected Kohn–Sham excitation spectrum matches well the spectra obtained in Marsusi et al. [22] using time-dependent DFT and the B3LYP functional. The two methods yield very similar excitation energies (within 0.2 eV) and oscillator strengths. Given the large broadening of ~1 eV that the quantum nuclear dynamics induces on the absorption spectra ( Fig. 2b ), this level of agreement is very satisfactory and motivates our use of a simple scissor-corrected DFT-LDA approach. Semiclassical optical absorption using ISMC In order to evaluate the integral over R in equation (1) and obtain the blue areas of Fig. 2b we proceeded as follows. We expressed the Cartesian coordinates R of the N nuclei in terms of the 3 N normal mode coordinates u i using the standard transformation , with R I β the position of nucleus I along the Cartesian direction β , R 0,I β the corresponding equilibrium coordinate, M I , m p the nuclear and proton masses, respectively, and e i , I β the components of the eigenvectors of the dynamical matrix. In the following, we use u as a shorthand for all the normal mode coordinates u i , and we refer to the above coordinate transformation as R = T [ u ]. By defining and P ( u )=|Φ 0,0 ( T [ u ])| 2 we can rewrite equation (1) as: σ ( ω )=∫d uP ( u ) S ( ω ; u ). The six modes corresponding to translations and rotations of the system do not contribute to the integral and were omitted. In the normal mode coordinates, the ground-state nuclear wavefunction Φ 0,0 ( u ) is a product of gaussians within the harmonic approximation, therefore P ( u ) is a proper probability distribution and can be used as the importance function in ISMC. The integral over u was evaluated using ISMC as the average σ( ω )=‹ S ( ω ; u )› MC , where each configuration u was drawn from a random sample distributed according to the importance function P ( u ). In this procedure for each set of normal coordinates u we generated a new nuclear configuration R = T [ u ], and calculated the corresponding DFT optical spectum S ( ω ; u ). The average was obtained by accumulating the contributions of many Monte Carlo steps. Supplementary Fig. S2 shows the convergence of this procedure with the number of Monte Carlo steps by comparing the optical spectra of adamantane calculated with 500 and 10,000 configurations, respectively. The lineshape is essentially converged with only 500 steps, and the residual noise arises from our choice of binning each contribution into very fine energy intervals. Supplementary Fig. S2 also shows that if we introduce a Lorentzian broadening of 50 meV, the variation between the two lineshapes is very small. The rapid convergence of our procedure stems from the use of importance sampling. Constrained-LSDA vertical and adiabatic excitations In Fig. 2b we compared the excitation energies of the fundamental optical transition calculated in the vertical approximation and in the adiabatic approximation. In both cases the excitation energies were evaluated as the sum of total energy differences and the empirical scissor correction discussed above. The total energy differences between ground and excited states were calculated using a constrained local spin-density approximation to DFT (C-LSDA). The choice of C-LSDA was motivated by previous investigations showing that this approximation yields excited-state geometries in good agreement with the more sophisticated Bethe–Salpeter approach [48] . Group-theoretical considerations indicate that the fundamental neutral excitations of adamantane (point group T d ) and triamantane (point group C 2 v ) are HOMO–LUMO transitions, T 2 → A 1 for adamantane and B 2 → A 1 for triamantane. In diamantane (point group D 3 d ), the A 1 g → A 1 g transition between the HOMO and LUMO is forbidden, therefore the first allowed transition is from the HOMO to the LUMO+1, A 1 g → A 2 u . Following these observations, we considered singlet excitations whereby one electron is promoted from HOMO to LUMO (adamantane and triamantane) or to LUMO+1 (diamantane) by constraining the occupation numbers of the Kohn–Sham states. The vertical transition energy was calculated as E v = E s ( R 0 )− E 0 ( R 0 ), with E 0 ( R 0 ) and E s ( R 0 ) the total energies of the ground and singlet excited states, respectively, both evaluated at the equilibrium nuclear geometry R 0 of the electronic ground state. The adiabatic excitation energy corresponds to a transition between the zero-phonon lines in the ground and excited states, and is given by: . In this expression, R s indicates the equilibrium nuclear geometry in the excited singlet state, and ω 0, i and ω s , i are the vibrational frequencies in the ground and excited states, respectively. The adiabatic excitation energy is decomposed in three contributions: the vertical transition E v , the structural relaxation upon photoexcitation E rel = E s ( R s )− E s ( R 0 ), and the change in zero-point energy , in such a way that E a = E v + E rel + E zpe . We calculated E v =5.93 eV, E rel =−0.33 eV, E zpe =−0.32 eV for adamantane, E v =6.20 eV, E rel =−0.28 eV, E zpe =−0.27 eV for diamantane, and E v =5.36 eV, E rel =−0.24 eV, E zpe =−0.25 eV for triamantane. ISMC evaluation of Condon integrals In Fig. 2a , we presented the optical absorption spectrum of adamantane calculated using the Franck–Condon approximation of equation (2). In the Frank–Condon approach, the lowest-energy optical excitations correspond to the vibronic transitions between the ground state and the excited singlet state whose energies are given by: with the occupation numbers of the vibronic state ν. Near the absorption onset the dipole matrix element is approximated by a constant. The demanding part of the calculation is the evaluation of the Condon integrals ∫d R Φ s ,ν ( R )Φ 0,0 ( R ) for all possible final vibronic states ν [49] . As the number of vibronic states increases combinatorially with excitation energy, we restricted the sum over final states to six vibrational modes (C–C–C deformation modes at 56.2 and 82.0 meV; C–C stretch modes at 95.8 meV; C–H rock and C–C stretch mode at 110.2 meV; C–C stretch modes at 128.6 and 149.4 meV [50] ), and we considered occupations numbers with up to three phonons in each mode, , yielding a total of 4,096 final states. These six vibrational modes were selected on the grounds that they provide the largest contribution to the absorption spectrum when only one-phonon excitations are considered. In order to evaluate Condon integrals the initial and final states Φ 0,0 and Φ s ,ν are expressed in the normal mode coordinates as products of gaussians. We note that the normal coordinates in the ground and excited states do not coincide owing to the change in the equilibrium geometry and dynamical matrix upon photoexcitation (Duschinsky effect). We calculated Condon integrals using ISMC. In this case, the importance function is taken to be P ( u )=Φ 0,0 ( u )/ Z , with the normalization factor Z =∫d u Φ 0,0 ( u ). The function P is a proper probability distribution as the ground-state nuclear wavefunction Φ 0,0 is nodeless. Other choices for the importance function are possible, for example, . Our choice Φ 0,0 has the advantage that it samples the tails of the wavefunction correctly. Similarly to the case of the semiclassical Franck–Condon approximation, we evaluate Condon integrals as a Monte Carlo average: ∫d R Φ s,ν ( R )Φ 0,0 ( R )= Z ‹Φ s ,ν ( u s [ u ])› MC . In this expression u s [ u ] stands for the set of normal mode coordinates in the reference frame of the singlet excited state, which yield the same atomic positions as the normal mode coordinates u in the ground state. The link between u and u s is given by two subsequent coordinate transformations u → R and R → u s . The function Φ s,ν ( u s [ u ]) to be evaluated at each Monte Carlo step is obtained as a product of harmonic oscillator wavefunctions specified by the occupation numbers . In this procedure, the misalignment of the nuclear wavefunctions in the ground and excited state makes the convergence of the ISMC procedure more demanding than for the semiclassical Franck–Condon approximation, for example, the calculation of the adiabatic transition in adamantane to an accuracy of 0.1% requires 200 million Monte Carlo steps. F.G. conceived the project. C.E.P. performed the calculations and data analysis. Both authors developed the theoretical framework, discussed the results and wrote the manuscript. How to cite this article: Patrick, C. E. and Giustino, F. Quantum nuclear dynamics in the photophysics of diamondoids. Nat. Commun. 4:2006 doi: 10.1038/ncomms3006 (2013).